Evidence of an inhibitory restraint of seizure activity in humans The location and trajectory of seizure activity is of great importance, yet our ability to map such activity remains primitive. Recently, the development of multi-electrode arrays for use in humans has provided new levels of temporal and spatial resolution for recording seizures. Here, we show that there is a sharp delineation between areas showing intense, hypersynchronous firing indicative of recruitment to the seizure, and adjacent territories where there is only low-level, unstructured firing. Thus, there is a core territory of recruited neurons and a surrounding 'ictal penumbra'. The defining feature of the 'ictal penumbra' is the contrast between the large amplitude EEG signals and the low-level firing there. Our human recordings bear striking similarities with animal studies of an inhibitory restraint, indicating that they can be readily understood in terms of this mechanism. These findings have important implications for how we localize seizure activity and map its spread. The recruitment of cortical territories to a seizure is one of the most important brain state transitions: it represents the difference between information processing through normal pathways and activity spreading in a pathological and escalating manner. Animal research has consistently shown two characteristic electrographic hallmarks of an established seizure, namely the paroxysmal depolarizing shift recorded in individual cells [1] , [2] , [3] , [4] and hypersynchronous discharges recorded across populations [5] . These features are consistent with the large amplitude signals apparent in clinical EEG records, yet surprisingly, several studies of unit activity in humans have failed to find evidence of these 'signature' events [6] , [7] , [8] , even within the 'epileptogenic zone', the presumptive site of origin of the seizure. These recent human studies, thus, call into question much of our understanding of epilepsy derived from animal work. A critical issue to consider here, however, is how we localize seizure activity. This is important not just for how we interpret these human unit recordings, but also for clinical practice. One of the few treatment options available to patients with pharmacoresistant focal epilepsy is to identify the brain area from which seizures arise and remove it. As the risks to the patient from such a procedure are substantial, it is necessary to define the epileptogenic zone as accurately as possible [9] . Key localizing information should be available from subdural EEG recordings, but animal studies suggest that there may be a major pitfall in how EEG recordings are interpreted. Studies of epileptiform propagation in mouse brain slices clearly show territories ahead of the ictal wavefront where there are very large amplitude excitatory and inhibitory conductances, with little postsynaptic recruitment [10] , [11] , [12] . Similar patterns have also been recorded in vivo , in animals following focal injection of GABA A antagonists [13] , [14] , [15] , [16] . The ictal wavefront generates huge feedforward excitation, yet a rapid feedforward inhibition provides a powerful restraint. We hypothesized, therefore, that if such a restraint also is present in naturally occurring (clinical) epilepsy, there should exist a 'penumbra' around the ictal activity where there are large amplitude EEG signals, reflecting feedforward synaptic currents, but with little actual local recruitment of neurons. It will be important to identify sites where large EEG signals do not correspond to local firing, because this may confound how we localize seizures. To examine this hypothesis, it is necessary to map out actual firing patterns over spatially extended territories during seizures and contrast this with the spread of postsynaptic currents away from the ictal focus. This has recently become possible following the development of microelectrode arrays (MEAs) suitable for use in humans [17] , [18] , [19] , [20] . Here, we present a series of MEA recordings, to show the spatial pattern of hypersynchronous recruitment of neurons to clinical seizures. We further characterize activity patterns in the surrounding territories, where there is a marked discrepancy between the large amplitude, low-frequency, extracellular signal indicative of large synaptic barrages and the low level of postsynaptic firing. Our recordings, therefore, show that the same features that define the restraint of cortical recruitment in simple animal models are present in vivo , in humans. Failures of propagation in an animal in vitro seizure model Full ictal recruitment in animal models seems to involve every neuron in the local cortical territory [10] , [21] , discharging at intense rates [1] , [22] . The 0 Mg 2+ model provokes slowly propagating events, where recruitment of new cortical territories is delayed by feedforward inhibition [10] , [12] . This inhibitory restraint has a characteristic electrophysiological signature in voltage clamp recordings of layer 5 pyramidal cells held at −30 mV (approximately half way between the glutamatergic and GABAergic reversal potentials). The key feature is a regular rhythm of predominantly inhibitory barrages, which matches the same rhythm of ictal discharges in the adjacent territory [10] , thus indicating that the ictal discharges are driving the rhythm. The voltage clamp recordings switch polarity when the ictal event invades the local territory [10] ; examples are shown in the last three upper traces in Fig. 1a . 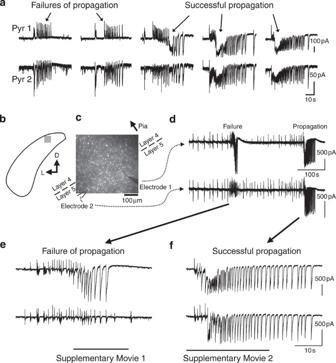Figure 1: Failure of propagation of full ictal events in mouse brain slices. (a) Five successive ictal events (shown left to right) recorded in two layer 5 pyramidal cells (PCs) 600 μm apart. Only in the last three events, does PC 1 make the transition from inhibitory to excitatory barrages, which is indicative of being incorporated into the ictal event. A very important point arising from a previous study10is that the upward deflections are not purely inhibitory, merely predominantly so. The level of inhibition simply occludes the very large concurrent excitatory drive at this time, which can be seen instead if the cell is clamped close to the GABAergic reversal potential. (b–f) Another example of δ-frequency, interictal-like activity, with concurrent low magnification Ca2+network imaging. The more extended field of view allows us to visualize the failure of propagation, as the view incorporates territories that are recruited to the ictal event and other regions that resist recruitment. (b) Schematic showing the field of view in the brain slice. (c) Field of view; the two electrodes are visible, located in layer 5. (d) Eight minute recording showing two full ictal events, the first of which is only manifest as δ-frequency interictal activity in electrode 2. (e,f) Detailed views of the two ictal events, showing the time period of two Ca2+network imaging movies (Supplementary Movies 1 and 2). Figure 1: Failure of propagation of full ictal events in mouse brain slices. ( a ) Five successive ictal events (shown left to right) recorded in two layer 5 pyramidal cells (PCs) 600 μm apart. Only in the last three events, does PC 1 make the transition from inhibitory to excitatory barrages, which is indicative of being incorporated into the ictal event. A very important point arising from a previous study [10] is that the upward deflections are not purely inhibitory, merely predominantly so. The level of inhibition simply occludes the very large concurrent excitatory drive at this time, which can be seen instead if the cell is clamped close to the GABAergic reversal potential. ( b – f ) Another example of δ-frequency, interictal-like activity, with concurrent low magnification Ca 2+ network imaging. The more extended field of view allows us to visualize the failure of propagation, as the view incorporates territories that are recruited to the ictal event and other regions that resist recruitment. ( b ) Schematic showing the field of view in the brain slice. ( c ) Field of view; the two electrodes are visible, located in layer 5. ( d ) Eight minute recording showing two full ictal events, the first of which is only manifest as δ-frequency interictal activity in electrode 2. ( e , f ) Detailed views of the two ictal events, showing the time period of two Ca 2+ network imaging movies ( Supplementary Movies 1 and 2 ). Full size image We now present other instances of sustained, predominantly inhibitory synaptic barrages that did not progress ( Fig. 1 ). Prolonged (>30 min) patch clamp recordings of multiple layer 5 pyramidal neurons showed such 'non-progressing' events in 26 out of 66 brain slices. Paired recordings often indicated full ictal activity, at the same rhythm, just a few hundred microns away ( Fig. 1 ), evidence of a highly localized failure of propagation. We further visualized this failure of propagation in five slices with network Ca 2+ imaging, with simultaneous paired voltage clamp recordings of pyramidal cells. Low magnification views clearly showed the sharp delineation of activity between territories that are participating in an ictal event and those that resist recruitment ( Fig. 1b ; Supplementary Movies 1 and 2 ). Higher magnification Ca 2+ imaging ( Fig. 2 ; Supplementary Movies 3 and 4 ) showed that even when a full ictal event fails to propagate, it still influences activity, because at the point of failure of propagation, neuronal activity was significantly increased above baseline levels (in the illustrated example, population average baseline activity (65 cells, 10 s periods)=4.97% (range 1.03–10.6%); activity during ictal failure=11.7% (4.70–22.3%); average during ictal event=53.8% (29.7–78.0%); and signals for individual cells were all normalized to their peak signal during the ictal event (100%), Fig. 2a ). Importantly though, there was only a low level of coherence between Ca 2+ signals in individual neurons, indicating that collectively, neurons were not conforming to the rhythm imposed by the ictal activity in the adjacent cortical territories. Similar patterns were also seen in three other slices in which we recorded very long periods (>15 s) of preictal activity before the ictal wavefront invaded the imaged field of view. In contrast, when territories were recruited to the event, every cell locally showed the same rhythmic discharges, reflected in a highly significant increase in coherence between cells ( Fig. 2e ). 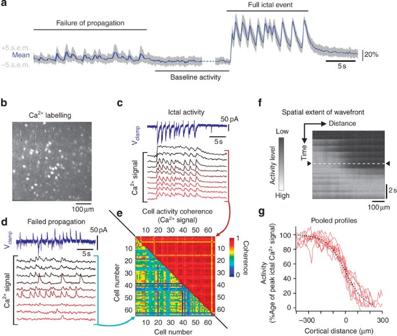Figure 2: Ca2+network imaging of failure of ictal propagation in mouse cortical slices. (a) Mean neuronal Ca2+fluorescence (centre-surround subtraction10) from 65 cells during three different epochs (epochs defined from concurrent voltage clamp recording of a layer 5 pyramidal cell within the field of view; all imaged cells within 200 μm of the recorded cell). Epoch 1 was a period of ictal activity elsewhere in the slice, which failed to invade the local territory. Epoch was baseline activity, and epoch 3 shows a full ictal event that did recruit the field of view. The grey shaded area shows the upper and lower extent of 5 s.e.m. signal for the 65 cells. Note: how even during the 'Failure of propagation', the mean signal comfortably exceeds baseline (mean±5× s.e.m.). (b) Brain slice loaded with OGB1. Two movies of this slice are in theSupplementary Information, showing a full ictal event and another event that failed to propagate into this territory. Representative traces of neuronal activity for these two events are shown incandd, together with a voltage clamp recording of a local pyramidal cell (Vhold=−30 mV). In the Vclamprecording, note the upward deflections (predominant inhibition) for the failure, and the downward deflections for the successful propagation, as shown also in the example in panela. (e) Coherence matrix for the Ca2+signal of 65 imaged neurons, showing a general lack of coherence when the ictal event fails to invade, in contrast with the highly coherent signal when the ictal event does invade (number of coherence measures=2080; non-participation coherence (mean±s.d.)=0.494±0.172; post-recruitment coherence=0.914±0.075;ts=102.0;P<<0.001, Student'st-test). (f) Line scan of a propagating ictal wavefront, derived from ×10 magnification Ca2+network imaging. Spatial profiles of the wavefront (dotted line) were derived during periods of stability. (g) The spatial profile of activity measured in eight brain slices. Figure 2: Ca 2+ network imaging of failure of ictal propagation in mouse cortical slices. ( a ) Mean neuronal Ca 2+ fluorescence (centre-surround subtraction [10] ) from 65 cells during three different epochs (epochs defined from concurrent voltage clamp recording of a layer 5 pyramidal cell within the field of view; all imaged cells within 200 μm of the recorded cell). Epoch 1 was a period of ictal activity elsewhere in the slice, which failed to invade the local territory. Epoch was baseline activity, and epoch 3 shows a full ictal event that did recruit the field of view. The grey shaded area shows the upper and lower extent of 5 s.e.m. signal for the 65 cells. Note: how even during the 'Failure of propagation', the mean signal comfortably exceeds baseline (mean±5× s.e.m.). ( b ) Brain slice loaded with OGB1. Two movies of this slice are in the Supplementary Information , showing a full ictal event and another event that failed to propagate into this territory. Representative traces of neuronal activity for these two events are shown in c and d , together with a voltage clamp recording of a local pyramidal cell (V hold =−30 mV). In the V clamp recording, note the upward deflections (predominant inhibition) for the failure, and the downward deflections for the successful propagation, as shown also in the example in panel a . ( e ) Coherence matrix for the Ca 2+ signal of 65 imaged neurons, showing a general lack of coherence when the ictal event fails to invade, in contrast with the highly coherent signal when the ictal event does invade (number of coherence measures=2080; non-participation coherence (mean±s.d. )=0.494±0.172; post-recruitment coherence=0.914±0.075; t s =102.0; P <<0.001, Student's t -test). ( f ) Line scan of a propagating ictal wavefront, derived from ×10 magnification Ca 2+ network imaging. Spatial profiles of the wavefront (dotted line) were derived during periods of stability. ( g ) The spatial profile of activity measured in eight brain slices. Full size image We can thus clearly distinguish between cortical areas that are being influenced by an ongoing seizure (receiving synaptic barrages emanating from the ictal focus, but with little local firing) and those areas that are fully participating. In non-recruited territories, there is an extreme disparity between the intensity of synaptic currents and the low level (relative to ictal firing), and low synchronization, of local neuronal firing. We assessed the boundaries of ictal activity by deriving the spatial gradients of the step function at the ictal wavefront from low-magnification Ca 2+ imaging (X4 or X10 objectives). We derived horizontal line scans of Ca 2+ signal within infragranular cortex [10] , first normalizing the baseline signal, and second, normalizing the range between quiescent baseline (0%) and maximal ictal activity (100%). The 20–80% rise of a propagating ictal wavefront measured 129.9±52.8 μm (mean±s.d. ; n =8). Differentiating pre- and post-recruitment states in humans Does this same separation of synaptic and firing activity also occur in spontaneous seizures in humans? We addressed this by examining spatio-temporal patterns of synaptic and unit activity during recruitment, and ahead of the ictal wavefront. These two facets of neuronal activity may be largely dissociated using bandpass filtering of extracellular recordings: the 2–50 Hz signal is dominated by the huge, rhythmic synaptic currents [10] , [22] (the lower frequency limit of 2 Hz excludes slower, non-synaptic currents, whereas the upper 50 Hz limit still incorporates the signals that dominate the electrographic signature of focal seizures), whereas very high-frequency (300 Hz–3 kHz) activity is considered to reflect unit activity. Future studies will address the intermediate frequency range between 50 and 300 Hz, which may also provide seizure localizing information [23] , [24] , but which typically has been studied with microwires or depth electrodes. We sampled a 4×4 mm cortical region with a dense MEA aligned with the clinical video EEG recording, allowing us to match low-frequency signals recorded from the MEA with those recorded from adjacent subdural electrodes ( Fig. 3 ). We looked for territories showing prominent rhythmic ictal discharges in the 2–50 Hz data but little unit activity, as seen in our in vitro studies ( Figs 1 and 2 ). 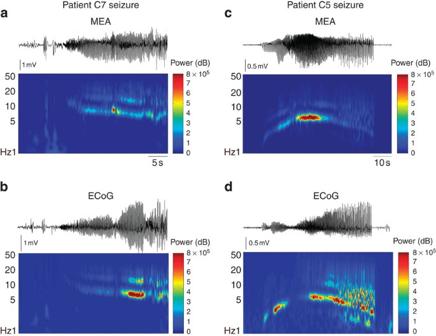Figure 3: Simultaneous MEA and EEG seizure recordings share common features in the EEG frequency range. (a,b) Patient C7 initiation, as recorded from one MEA channel (a) and the nearest active EEG channel (b, electrode 22,Supplementary Fig. 1). Spectrograms computed using the Morlet wavelet transform (1–50 Hz) together with the filtered time series signal are shown. This seizure followed the most common neocortical onset pattern, reflected in both the MEA and EEG channels, with an initial epileptiform discharge followed by rhythmic beta activity that gradually slows to the theta range and gains in amplitude. The seizures recorded from patients C2, C3 and C4 followed this same general pattern. (c,d) Simultaneous MEA and adjacent EEG recordings from patient C5. This seizure, following an electrographic pattern that is less common but still well known in neocortical EEG recordings, was characterized by an initial monomorphic delta rhythm that gradually increased in frequency to the theta range, then slowed to a 3–4-Hz spike and wave rhythm before offset. Figure 3: Simultaneous MEA and EEG seizure recordings share common features in the EEG frequency range. ( a , b ) Patient C7 initiation, as recorded from one MEA channel ( a ) and the nearest active EEG channel ( b , electrode 22, Supplementary Fig. 1 ). Spectrograms computed using the Morlet wavelet transform (1–50 Hz) together with the filtered time series signal are shown. This seizure followed the most common neocortical onset pattern, reflected in both the MEA and EEG channels, with an initial epileptiform discharge followed by rhythmic beta activity that gradually slows to the theta range and gains in amplitude. The seizures recorded from patients C2, C3 and C4 followed this same general pattern. ( c , d ) Simultaneous MEA and adjacent EEG recordings from patient C5. This seizure, following an electrographic pattern that is less common but still well known in neocortical EEG recordings, was characterized by an initial monomorphic delta rhythm that gradually increased in frequency to the theta range, then slowed to a 3–4-Hz spike and wave rhythm before offset. Full size image In all subjects, the array was located within the presumptive neocortical 'seizure onset zone' defined by conventional clinical methods [9] (see Supplementary Information ; we discuss, later, the validity of the term 'seizure onset zone'). Despite this placement, our recordings did not encompass the initiating event but rather gave us a detailed view of early seizure propagation. Seven subjects were implanted, but no seizures were recorded in two, so we limit our description to the remaining five (72 complex partial seizures; Supplementary Table S1 ). The multiunit activity recorded in the MEAs showed two distinct patterns: seizures that invaded the MEA territory (patients C2, C5 and C7; Figs 4 and 5 ) and those that did not (C3 and C4; Fig. 6 ). In two patients (C5 and C7), the multiunit activity clearly showed the ictal wavefront as it progressed across the MEA ( Fig. 4 ; Supplementary Movie 5 ). These are the first recordings of hypersynchronous neuronal recruitment, visualized as unit activity, over extended spatial territories in vivo , in humans. 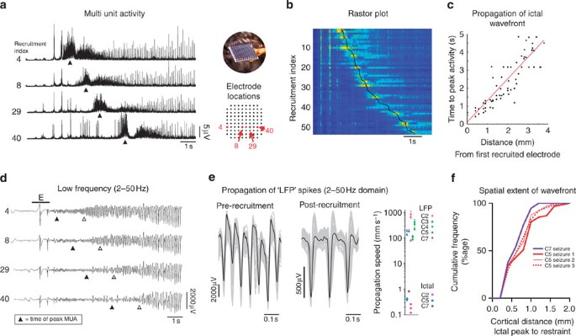Figure 4: Seizure propagationin vivoin a human. (a) Multiunit activity in four electrodes, spaced at 800 μm intervals in patient C7, showing the spatial progression of the ictal wavefront and illustrating the pre-recruitment, recruitment and post-recruitment seizure phases. Black arrowheads denote the progression of the ictal wavefront, and delineate the pre-recruitment from the post-recruitment period. The recruitment index refers to the temporal ordering according to the time of the sharp increase in firing ('recruitment'). Inset: layout schematic showing the locations of the four selected channels, with the convention that the wire exits on the left. (b) Raster plot showing the colour-coded multiunit activity for all electrodes in C7, which showed unit activity ('hot' colours active; 'cold' colours inactive), ordered according to the time of recruitment. (c) The delay in electrode recruitment plotted versus the distance from the first recruited (index) electrode. The slope of the line of best fit indicates a propagation speed of 0.83 mm s−1. (d) Low-frequency (2–50 Hz) signal from the same electrodes shown in panela. Note the absence of any visually notable features in this bandwidth that correspond with the clear recruitment process in the multiunit activity (filled arrowheads), although note also that the transition into the clonic phase (open arrowheads) corresponds to an increase in amplitude that can be seen as a delayed progression. (e) Overlays of the 2–50 Hz signal recorded at all microelectrodes for short periods before and after recruitment. Note: the smear of signals, due to propagation across the array, and also the relatively greater degree of pre-recruitment variability compared with post-recruitment. Propagation of these events was consistent in different subjects, and over 2 orders of magnitude (>100×) faster than ictal wavefront propagation. This 100-fold difference in propagation speed mirrors exactly the situation in the 0 Mg2+model27where forward and backward projecting synaptic barrages that propagate with identical speeds, roughly 100-fold faster than the ictal wavefront. (f) Estimates of the spatial extent of the wavefront. For the time of peak ictal activity in each individual electrode, we plot the distribution of distances to the nearest pre-recruitment electrode (see Methods for further detail). Figure 4: Seizure propagation in vivo in a human. ( a ) Multiunit activity in four electrodes, spaced at 800 μm intervals in patient C7, showing the spatial progression of the ictal wavefront and illustrating the pre-recruitment, recruitment and post-recruitment seizure phases. Black arrowheads denote the progression of the ictal wavefront, and delineate the pre-recruitment from the post-recruitment period. The recruitment index refers to the temporal ordering according to the time of the sharp increase in firing ('recruitment'). Inset: layout schematic showing the locations of the four selected channels, with the convention that the wire exits on the left. ( b ) Raster plot showing the colour-coded multiunit activity for all electrodes in C7, which showed unit activity ('hot' colours active; 'cold' colours inactive), ordered according to the time of recruitment. ( c ) The delay in electrode recruitment plotted versus the distance from the first recruited (index) electrode. The slope of the line of best fit indicates a propagation speed of 0.83 mm s −1 . ( d ) Low-frequency (2–50 Hz) signal from the same electrodes shown in panel a . Note the absence of any visually notable features in this bandwidth that correspond with the clear recruitment process in the multiunit activity (filled arrowheads), although note also that the transition into the clonic phase (open arrowheads) corresponds to an increase in amplitude that can be seen as a delayed progression. ( e ) Overlays of the 2–50 Hz signal recorded at all microelectrodes for short periods before and after recruitment. Note: the smear of signals, due to propagation across the array, and also the relatively greater degree of pre-recruitment variability compared with post-recruitment. Propagation of these events was consistent in different subjects, and over 2 orders of magnitude (>100×) faster than ictal wavefront propagation. This 100-fold difference in propagation speed mirrors exactly the situation in the 0 Mg 2+ model [27] where forward and backward projecting synaptic barrages that propagate with identical speeds, roughly 100-fold faster than the ictal wavefront. ( f ) Estimates of the spatial extent of the wavefront. For the time of peak ictal activity in each individual electrode, we plot the distribution of distances to the nearest pre-recruitment electrode (see Methods for further detail). 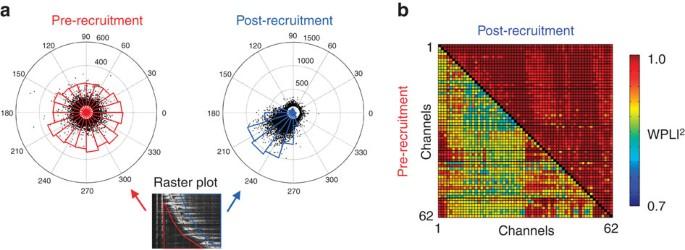Figure 5: Hypersynchronous activity and electrode coherence following recruitment. (a) Action potential—field potential phase plots showing a marked transition in the phase timing of action potentials, from the pre-recruitment phase when action potentials occur with equal probability at all phases of the field potential, to the post-recruitment period when firing phase is very skewed, indicating that firing is strongly influenced by the rhythm of the seizure. (b) The low frequency (2–50 Hz) signature of ictal invasion is a dramatic increase in phase coherence between electrodes (WPLI, weighted phase lag index, pairedt-test,T=83.87,P0.001,n=165). Full size image Figure 5: Hypersynchronous activity and electrode coherence following recruitment. ( a ) Action potential—field potential phase plots showing a marked transition in the phase timing of action potentials, from the pre-recruitment phase when action potentials occur with equal probability at all phases of the field potential, to the post-recruitment period when firing phase is very skewed, indicating that firing is strongly influenced by the rhythm of the seizure. ( b ) The low frequency (2–50 Hz) signature of ictal invasion is a dramatic increase in phase coherence between electrodes (WPLI, weighted phase lag index, paired t -test, T =83.87, P 0.001, n =165). 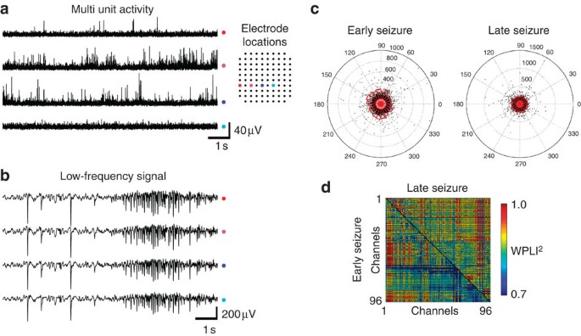Figure 6: Electrophysiological indicators of non-participating cortical territories in human seizures. (a) Multiunit activity and (b) 2–50 Hz signal during a seizure in patient C4. Although some electrodes clearly show firing activity, this was at a low level, with no obvious spatial pattern or wave of recruitment. (c) Action potential—field potential phase plots showing that the firing phase of the units remains in the 'pre-recruitment' pattern throughout the event, at no time showing any significant phase angle preference (note different radial scales in early and late seizures). (d) The inter-electrode coherence measure shows a minimal increase from early to late seizure periods, in marked contrast to the striking increase in coherence associated with ictal invasion of the MEA territory (seeFig. 5b). Full size image Figure 6: Electrophysiological indicators of non-participating cortical territories in human seizures. ( a ) Multiunit activity and ( b ) 2–50 Hz signal during a seizure in patient C4. Although some electrodes clearly show firing activity, this was at a low level, with no obvious spatial pattern or wave of recruitment. ( c ) Action potential—field potential phase plots showing that the firing phase of the units remains in the 'pre-recruitment' pattern throughout the event, at no time showing any significant phase angle preference (note different radial scales in early and late seizures). ( d ) The inter-electrode coherence measure shows a minimal increase from early to late seizure periods, in marked contrast to the striking increase in coherence associated with ictal invasion of the MEA territory (see Fig. 5b ). Full size image The key observation was that in all electrodes, there was a marked discrepancy between the apparent onset time of the ictal rhythm in the low-frequency domain and the actual time when neurons were recruited, as indicated by the transition in the neuronal firing patterns. The earliest low-frequency ictal rhythms propagated rapidly across all MEA channels and as well the nearby ECoG channels ( Fig. 4f ; Supplementary Movie 5 . See also [25] ; note that these signals cannot reflect volume conduction, which would be seen instantaneously across all electrodes). At this time, however, there was only an irregular and relatively low level of unit activity, and the real recruitment, characterized by an intense sharp increase in unit activity that lasted about a second, occurred only later. The leading edge of the wavefront was sharply defined, with <1 mm from the wavefront peak to the pre-recruitment territory ( Fig. 4f ). On occasions, transient localized bursts of activity could be seen ahead of the wavefront, but these did not 'seed' or propagate from that locus at that time and were duly incorporated into the full ictal event by the subsequent progression of the wavefront. It is likely, however, that saltatory propagation through long axonal tracts occurs, but a far wider spatial sampling of unit firing would be required to detect this. The propagation speeds of the ictal wavefronts in C5 and C7 were calculated using the timing of maximal tonic firing in each electrode ( Fig. 4c ). Patient C2 was in partial status epilepticus throughout the recording period and did not show the same sudden recruitment pattern, instead showing surges of activity, which likewise, spread slowly across the MEA (five seizures; mean 0.18, range 0.12–0.26 mm s −1 ). These recordings show that seizures in vivo propagate with remarkable similarity to the slow ictal wavefronts in the in vitro 0 Mg 2+ model [10] , [12] , [26] (albeit, far slower than epileptiform clonic discharges recorded in this model [27] or epileptiform events recorded in disinhibited slices [28] , [29] , [30] , both of which propagate between 10 and 200 mm s −1 , but notably, both also represent instances where there is little or no effective feedforward inhibition to slow propagation). There are further clear parallels between in vivo and in vitro activity with regard to the spatially sharp drop in firing activity at the wavefront ( Figs 2g and 4f ) and the widely and rapidly distributed 2–50 Hz signal ( Fig. 4e ; this 2–50 Hz is comparable to the distribution of synaptic barrages seen in vitro [27] ), extending well beyond the wavefront. Indeed, the speed of the ictal wavefront was orders of magnitude slower than events recorded in the 2–50 Hz bandwidth ( Fig. 4e ). The presence of well-demarcated recruitment events allowed us to subdivide the seizure recordings from patients C5 and C7 into pre- and post-recruitment periods, and thus determine how activity patterns change at the time of recruitment. The pre-recruitment period was characterized by modest (<fivefold) increases in firing rate over baseline activity (Kruskal–Wallis test, P <0.01). Despite this evidence of local influence by the seizure, there was no significant phase relationship of unit firing to the 2–50 Hz signals recorded at the same electrode ( Fig. 5a ; bootstrap analysis, see Methods for details). In contrast, the firing rates during and after recruitment were much higher, up to 30 times the baseline rate, and following recruitment were tightly phase locked to the dominant low-frequency rhythm (bootstrap procedure; P <0.05; n =165 channels; Fig. 5a ). Notably, the peak firing occurred at the same field potential phase at the late seizure stage in all seizures examined in these patients (5, 3 and 1 seizures recorded from patients C2, C5 and C7, respectively). In patient C2, spikes were also significantly phase-locked to low-frequency activity in the early seizure stage, which may represent a special feature of status epilepticus. A particularly striking observation was that the transition to recruitment was not marked by any obvious change in the low-frequency signal (see filled arrowheads in Fig. 4a,d ), although the propagation of the wave was subtly evident in the waveform amplitudes as the ictal pattern progressed into the later, clonic phase (open arrowheads). It was notable, therefore, that other consistent indicators of recruitment may still be derived from the low-frequency signal: namely, a transient drop in non-zero phase coherence followed by a marked increase after recruitment (paired t -test, P <0.001; n =165 channels; Fig. 5b , Supplementary Table S2 and Supplementary Fig. S5A ). The change in coherence is readily apparent in overlays of the 2–50 Hz signals ( Fig. 4e ). Non-recruited territories In patients C3 and C4 ( Fig. 6 ), unit activity peaked at 3–4 times the baseline activity during seizures (10 seizures), and spiking showed no significant phase relationship to the large amplitude 2–50 Hz signals at any time throughout the seizure ( Fig. 6a ). Furthermore, unlike the simple spatial structure of the travelling wavefront seen in recruited territories, there was no obvious spatial arrangement of changes in activity across the array of electrodes. Also, there was a decrease in the inter-electrode coherence between the early and late seizure periods (paired t -test, P <0.001; n =612 channels; Fig. 5b , Supplementary Table S2 ). In all these features, the activity throughout the seizure corresponded to the pre-recruitment pattern seen in patients C5 and C7. The moderate increase in unit activity in C3 and C4 indicated that the MEA territories were clearly influenced by the ongoing seizure, but importantly, these territories did not display the expected hallmarks of a seizure: namely, the abrupt onset of tonic firing that heralds the arrival of the ictal wavefront or the intense, hypersynchronous firing that accompanies paroxysmal depolarizing shifts. We concluded, therefore, that as the activity seems identical to that recorded ahead of ictal waves in other subjects, the MEA territories in these two patients were not recruited to the seizure, but rather were in the ictal penumbra. This 'penumbral activity pattern' at the MEA in these two latter patients was a surprising finding, as MEAs in all patients were placed within the clinically identified 'seizure onset zone', where subdural electrodes consistently recorded large amplitude signals during seizures. Importantly, surgical outcomes were good when this zone was resected ( Supplementary Table S1 ), implying that the genuine seizure focus was indeed located within this territory. Therefore, the seizure onset zone, as it is usually defined, also encompasses areas that are only recruited with delay (patients C5 and C7) or resist recruitment into the seizure altogether (C3 and C4). The implication is that the brain volume that must be resected to control seizures is likely to be far smaller than is currently deemed necessary. Stereotypy in seizures A common clinical observation is that seizure semiology in individuals is conserved across repeated seizures, as is the electrographic (EEG) appearance. This was also the case in the four subjects in whom more than one seizure was recorded. In all four, the low-frequency electrographic patterns for individual patients were very stereotyped from seizure to seizure, both in the multi-electrode array and also in the subdural electrodes ( Fig. 7 ), even though the predominant frequency and the ictal evolution all differed between patients. Thus, stereotypy was also shown in the fine scale spatial structure of seizure activity. Together, these observations strongly suggest that core pathological neuronal firing is also spatially stereotyped from seizure to seizure. 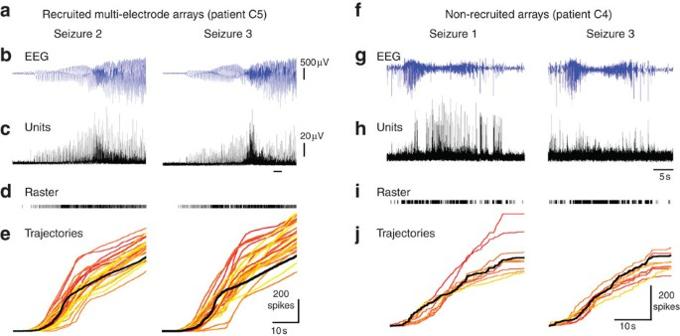Figure 7: Stereotyped firing patterns are another hallmark of territories that are recruited to seizures. (a) Recording from a single microelectrode implanted in a cortical area fully recruited into seizures (patient C5), showing LFP in the frequency range of clinical EEG in panelb, and multiunit activity in panelc. For clarity, only the initial portions of both seizures are shown. Note: the highly conserved field potential (panelb) and multiunit activity (c). Paneldshows units from a different channel, whileeshows the cumulative firing trajectories for every channel with a firing rate exceeding 12 spikes s−1. Trajectories were highly correlated across the three recorded seizures (Spearman coefficients 0.71±0.14 for 84 channels). The black line is the trajectory for the electrode raster ind, and the colours for other electrodes are preserved in the two plots for ease of comparison. (f) The same plots for a territory not incorporated into the seizure (patient C4). (g) We show recordings from the same electrode during two seizures. Note that the LFP pattern is again highly conserved, but the unit activity is not, as evident in both the single electrode examples (h,i) and also the high, seizure to seizure variability of trajectories (Spearman coefficients 0.38±0.26 for 30 channels across seven seizures) (j). Again we only show trajectories for electrodes showing greater than 12 spikes s−1during all seizures, and sojexcludes examples like that shown inh, which are even more extreme. Figure 7: Stereotyped firing patterns are another hallmark of territories that are recruited to seizures. ( a ) Recording from a single microelectrode implanted in a cortical area fully recruited into seizures (patient C5), showing LFP in the frequency range of clinical EEG in panel b , and multiunit activity in panel c . For clarity, only the initial portions of both seizures are shown. Note: the highly conserved field potential (panel b ) and multiunit activity ( c ). Panel d shows units from a different channel, while e shows the cumulative firing trajectories for every channel with a firing rate exceeding 12 spikes s −1 . Trajectories were highly correlated across the three recorded seizures (Spearman coefficients 0.71±0.14 for 84 channels). The black line is the trajectory for the electrode raster in d , and the colours for other electrodes are preserved in the two plots for ease of comparison. ( f ) The same plots for a territory not incorporated into the seizure (patient C4). ( g ) We show recordings from the same electrode during two seizures. Note that the LFP pattern is again highly conserved, but the unit activity is not, as evident in both the single electrode examples ( h , i ) and also the high, seizure to seizure variability of trajectories (Spearman coefficients 0.38±0.26 for 30 channels across seven seizures) ( j ). Again we only show trajectories for electrodes showing greater than 12 spikes s −1 during all seizures, and so j excludes examples like that shown in h , which are even more extreme. Full size image We therefore examined stereotypy in unit activity, by defining 'firing trajectories', cumulative frequency plots of unit activity recorded over the course of a seizure. All three seizures recorded in C5, and five seizures studied in C2, showed consistent recruitment patterns and strikingly similar multiunit firing trajectories in all electrodes ( Fig. 7a ; Supplementary Table S3 ). In contrast, non-recruitment throughout the seizure was observed consistently in C3 and C4, and multiunit activity at each electrode varied greatly from seizure to seizure ( Fig. 7f ). Thus, stereotypical firing is a further feature that differentiates between recruited and non-recruited activity patterns. There are two important conclusions from these observations. First, that very focal, stereotyped firing may also generate the far more spatially extended stereotypy in the low-frequency signal, presumably reflecting a wide distribution of postsynaptic currents. Conversely, low-frequency stereotypy does not necessarily reflect local stereotyped firing, but may arise from a far smaller focus located elsewhere. Recruitment is associated with homogeneous firing A previous study of implanted MEAs in focal human epilepsy reported an increased heterogeneity of firing during the seizure, shown by the Fano factor (variance of spiking divided by the mean; see Methods for further details) being persistently raised throughout the event [6] . To provide a direct comparison with our recordings, we repeated this analysis. In all seizures, the start of the event coincided with a large rise in the Fano factor ( Fig. 8 ), but once the ictal wavefront had incorporated, the entire MEA, the Fano factor, dropped sharply to below baseline levels (red arrows in Fig. 8a ). This drop was not seen in cases when the seizure failed to invade the MEA territory (that is, the MEA was located in the penumbral territory throughout). 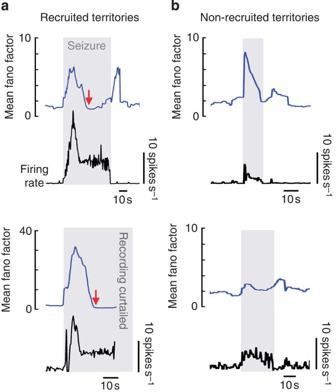Figure 8: Sharp drop in activity variance as wavefront incorporates cortical territories. (a) The Fano factor, a measure of firing heterogeneity, has been used previously to characterize neuronal spiking patterns during seizures6. In territories that are fully recruited to a seizure, the Fano factor increases sharply during the period when the ictal wavefront passes across the MEA, but once it has incorporated the entire array, the metric drops sharply to below baseline, even though firing rate remains very high (red arrows). (b) In territories that are penumbral to the seizure throughout its duration, the Fano factor remains persistently raised above baseline. Figure 8: Sharp drop in activity variance as wavefront incorporates cortical territories. ( a ) The Fano factor, a measure of firing heterogeneity, has been used previously to characterize neuronal spiking patterns during seizures [6] . In territories that are fully recruited to a seizure, the Fano factor increases sharply during the period when the ictal wavefront passes across the MEA, but once it has incorporated the entire array, the metric drops sharply to below baseline, even though firing rate remains very high (red arrows). ( b ) In territories that are penumbral to the seizure throughout its duration, the Fano factor remains persistently raised above baseline. Full size image We show the first spatially extended recordings of hypersynchronous recruitment to a seizure in humans. We further characterize activity patterns in the surrounding areas (the penumbra) that show only low, desynchronized firing, and which contrasts with the large amplitude, low-frequency signals recorded there. Moreover, there are clear parallels with animal research examining the protective inhibitory restraint opposing epileptic spread. The concept of an inhibitory restraint of spreading ictal activity derives from both in vivo [13] , [14] , [15] , [16] and in vitro animal studies [10] , [11] , [12] . These, however, are all 'acute' models of the disease process, so it is important to consider their relevance to the chronic phenotype seen in our patients with intractable epilepsy. The critical overlap is that even in these human subjects, seizure activity may impact on non-epileptogenic cortical territories. Indeed, the basic presumption underlying epilepsy surgery is that a focal pathology may be removed to leave just functional cortex. It is thus entirely reasonable that inhibitory restraint mechanisms recorded in acute models of epilepsy, induced pharmacologically in previously normal tissue, should resemble non-epileptogenic territories in humans that are being bombarded with synaptic barrages arising from a chronically pathological focus. It is important to recognize that even if surges of network activity may arise differently in acute and chronic epileptic foci, the response of surrounding tissue may still be the same. This study says little if anything about the initiation of the event, other than that it may be very focal, but does consider how activity invades new territories. The exact mechanism by which the restraint is overcome during recruitment remains to be determined, but may involve activity-dependent mechanisms that either boost excitatory neurotransmission [31] or compromise inhibitory neurotransmission [32] , [33] , [34] , or both. Translating animal findings to the human condition is difficult. Obviously, animal models allow many greater possibilities for research than human recordings, and our understanding of the inhibitory restraint reflects this: it is simply not possible to do patch clamp recordings or Ca 2+ imaging of spontaneous seizures in humans. The ability, though, to broadly separate synaptic currents from postsynaptic firing in extracellular microelectrode recordings using bandpass filters provides a key test of the inhibitory restraint hypothesis. Large, low-frequency (EEG) signals are indicative of large postsynaptic currents, and so a failure to detect postsynaptic firing locally provides strong support for our hypothesis. Further support is provided by similarities between animal and human recordings in terms of propagation speed, changes between pre- and post-recruitment activity with respect to the phase of firing, and changes in coherence of electrophysiological signals. Brain slice data shows clearly that ahead of the ictal wavefront there are very large feedforward excitatory and inhibitory synaptic barrages, but with little postsynaptic recruitment [10] , [12] . The implication from our human recordings is that exactly the same phenomenon occurs also in the human brain during epileptic propagation. Thus, ictal neuronal discharges trigger a rapid spread of postsynaptic currents away from the ictal wavefront via long axonal pathways. This rapid distribution of synaptic currents is evident in EEG recordings [35] , [36] , which therefore give the impression that seizure onset occurs simultaneously over broad, even multilobar, regions, when, in fact, these low-frequency ictal rhythms may be far from the location of the presynaptic discharging neurons. There is thus a 'penumbra' around the ictal activity, where there is large amplitude EEG signal, but relatively little, and desynchronized, firing. Importantly, only in areas fully incorporated into the seizure did we see the intense, synchronous discharges that are the expected signature of the paroxysmal depolarizing shift [1] , [37] . Previous studies in humans with microelectrodes [6] , [7] , [8] have noted a surprising absence of synchronous neural firing during seizures. A possible explanation for this failure to record hypersynchrony may be that genuine ictal recruitment occurs in far smaller territories than has previously been suspected. The rapid distribution of postsynaptic currents away from a small focus of activity, which is apparent as large amplitude EEG signals, requires great care when interpreting recordings, particularly with regard to whether unit activity is being recorded at the ictal focus or in the penumbra. Given the clear evidence for hypersynchronous firing seen in some of the subjects we studied, particular caution should be taken using spike-sorting algorithms, as full ictal recruitment is likely to induce changes in spike shapes during paroxysmal depolarizing shifts. A key issue for future study is how representative these first recordings of hypersynchronous activity in humans are. It is notable that even though there were differences in the recording location and electrographic seizure onset patterns between subjects, the distinctive penumbral pattern was recorded in four out of five (the fifth was in continual status, so may represent an unusual case), and three out of five (including the patient in status) showed the same pattern of fully recruited ictal activity, as defined previously in animal models. There is thus a broad consistency between animal and human data about these two patterns of activity that can be recorded during a seizure: ictal and penumbral. Might there be other seizure types, perhaps arising from lower levels of activity distributed over wide territories? This debate may be settled by considering stereotypy: if seizures show the same pattern of EEG signal from seizure to seizure, it seems highly likely that the underlying pathological firing will also show stereotypy, and indeed, we showed exactly this for fully recruited territories, but significantly, not within the ictal penumbra. In conclusion, we have shown that established ictal discharges may fail to invade adjacent territories, even though the synaptic bombardment of these areas is extremely intense. We were able to identify several characteristic signals, in both mouse and human data, which differentiated such failures of propagation from the genuine recruitment of cortical territories to a seizure. Recruited territories showed a stereotyped, large (up to ~30-fold) increase in unit activity followed by phase locking of firing to the dominant low-frequency signals, homogeneity of firing across the territory (low Fano factor) and a high-phase coherence between nearby recording sites. In contrast, territories in the ictal penumbra (pre-recruitment in C5 and C7, and the entire seizure duration in C3 and C4) show a much lower level of firing, no stereotyped firing patterns, heterogeneity of firing across the array, no phase locking and minimal change in electrode coherence. We also show that the EEG recordings, limited as they are to conveying postsynaptic potential activity, are likely to be misleading about the location of seizure activity. This warrants a substantial revision of how we interpret the low-frequency patterns seen in subdural and scalp EEG recordings. Slice preparation All animal handling and experimentation were done according to National Institutes of Health and UK guidelines. Acute brain slices were prepared from young (postnatal day 13–21) C56/Bl6 mice. The animals were anaesthetized with ketamine–xylazine (10 mg kg −1 ) and the brain was removed. Coronal slices, 350 μm thick, were cut using a Leica vibratome (Nussloch, Germany), and the slices were then incubated in artificial cerebrospinal fluid (ACSF) containing 1 mM Mg 2+ ions. (NaCl, 125; NaHCO 3 , 26; dextrose, 10; KCl, 3.5; CaCl 2 , 2; NaH 2 PO 4 , 1.26; MgSO 4 , 1). Dye loading and imaging Slices were bulk loaded with Oregon Green 488 Bapta 1 (OGB1)-AM ester as follows. OGB1-AM (50 μg vial, Invitrogen, Carlsbad, CA) was mixed with 8 μl DMSO and 2 μl pluronic acid F-127 solution (10% in DMSO, Invitrogen). Meanwhile, the slices were preincubated at 37 °C for 5 min in 3 ml ACSF with 8 μl Cremophor EL solution (0.5% in DMSO, Sigma, St Louis, MO). The OGB1/pluronic acid/DMSO mixture was then added and the slices incubated for a further 30–40 min. The final concentrations were ~12 μM OGB1-AM ester; 0.6% DMSO; 0.002% Cremophor EL; 0.01% Pluronic F-127. The slices were then placed back in normal ACSF for at least 30 min before transferring to the recording chamber. OGB1 imaging was performed on two different systems: a spinning disk confocal (Solamere, Salt Lake City, UT) mounted on an Olympus BX/50WI (Tokyo, Japan) upright microscope (equivalent systems at Columbia and Newcastle), and also an Olympus DSU fluorescence microscope (Newcastle). All three rigs gave qualitatively the same biological recordings. The tissue was illuminated with a 488-nM laser (Coherent, Santa Clara, CA), controlled through an acoustic-optical tunable filter or using conventional FITC filter set (Olympus DSU). Images were collected at 7.5–60 Hz with either (Columbia) a Stanford Photonics (Palo Alto, CA) Mega camera, and streamed to a raid drive (Atto Bioscience, Rockville, MD) using QED software (QED Software Solutions, Delta, British Columbia, Canada), or (Newcastle) Hamamatsu CM9100/13 cameras. Offline analysis of the images was performed using ImageJ (NIH) and in-house software. Cellular Ca 2+ signals were derived from movies taken using X10 (NA=0.3) and ×20 (NA=0.9) objectives. Somata were identified as previously described [38] , [39] , [40] . The neuropil signal was subtracted from the somatic signal to derive the 'centre-surround' signal, which we found to be a better indicator of the activity pattern of individual cells during intense network activity [10] . Coherence measures ( Fig. 2e ) were done on the centre-surround signal. After Ca 2+ imaging, the slice was bathed briefly in sulforhodamine (SR101, Invitrogen; 3 ml of 1 μM solution (in ACSF), and subsequently washed through for at least 15 min) to label the astrocyte population [41] . The SR101 was visualized using epifluorescence illumination (rhodamine filter set). Electrophysiology Electrophysiological data were collected either using a Heka Elektronik (Lambrecht/Pfalz, Germany) EPC10 amplifier with Patchmaster software (Columbia) or Multiclamp 700B (Axon Instruments) (Newcastle). The bath was mounted on a Scientifica (Uckfield, East Sussex, UK) movable top plate fitted with a heater plate (Warner Instruments, Hamden, CT), and the incoming solution (perfusion at 1–3 ml min −1 ) was heated by a sleeve heater element (Warner Instruments). All imaging and electrophysiological recordings were done at 33–37 °C. Whole cell patch clamp recordings were made using 3–7 MΩ pipettes (borosilicate glass, Harvard; MX130 hydraulic micromanipulators, SD Instruments). The pipette solution contained 125 mM K methyl-SO 4 ; 10 mM K-Hepes; 2.5 mM Mg-ATP; 6 mM NaCl; 5 mM QX-314 ( N -(2,6-dimethylphenylcarbamoylmethyl)triethylammonium bromide), Tocris Bioscience, Ellisville, MO); 0.3 mM Na-GTP; 0.5% biocytin (weight/volume). For current clamp (I clamp ) recordings of action potential trains, the QX-314 was omitted. The electrophysiological data was analyzed offline using Igor (Wavemetrics, Lake Oswego, OR). There were no qualitative differences between the recordings from OGB1-loaded versus unloaded slices. Cells were routinely filled with biocytin during the recordings, and all slices were fixed and stained for biocytin. From the location of the stained cells, one could accurately determine which cortical laminae were imaged during the experiments. Human studies The study was conducted under the oversight of the Columbia University's Institutional Review Board and complied with all regulations. Adults with pharmacoresistant focal epilepsy undergoing chronic invasive EEG studies, in whom sublobar seizure onset localization was indicated by the presurgical evaluation, were eligible to participate. A 96-microelectrode, 4 mm×4 mm array designed to record from layers 4 and 5 (Neuroport, Blackrock Microsystems Inc., Salt Lake City, UT) [17] , [18] , [19] was implanted along with standard clinical sensors for the duration of the invasive evaluation. The implant site was selected to fall within the putative seizure onset zone and away from eloquent brain areas, to ensure that the site would be targeted for subsequent surgical treatment. Further details are presented in the Supplementary Online Material . Recording methods MEA signals were acquired continuously at 30 kHz per channel (0.3 Hz–7.5 kHz bandpass, 16-bit precision, range ±8 mV). Reference was either subdural or epidural, chosen dynamically based on recording quality. Subdural EEG signals were acquired using a standard clinical video EEG system (XLTek, Natus Medical Inc., Oakville, ON, Canada) at 500 Hz per channel (0.5–125 Hz bandpass, 24-bit precision). The two data sets were aligned by a pulse-coded signal delivered simultaneously to digital inputs of both recording systems. Seizures were identified first by the treating physicians in accordance with standard clinical practice, including a visual review of the XLTek recording, followed by subsequent reviews by two neurophysiologists (C.A.S. and R.G.E.). Data processing The first seizures (if available) from each patient were selected for detailed analysis, to avoid biasing the data set from the two patients where many seizures were recorded. Raw MEA signals were bandpass filtered (symmetric 500th order FIR) into LFP (2–50 Hz) and multiunit activity (300 Hz–3 kHz) data streams. LFP and multiunit activity were visually reviewed to exclude channels and time periods with excessive artefact. Spikes were detected from multiunit activity by identifying peaks with amplitude more than 4 s.d. above or below the mean for each data sample. Calculations were performed using in-house software (Matlab, Mathworks, Natick, MA). Identification of ictal wavefront The time of recruitment in each channel was determined by binning the detected spikes into 20 ms intervals and identifying the maximum peak. From this peak, we then calculated the distance to the nearest electrode with unit activity within 1 s.d. of the pre-recruitment mean. Wavefront speed was determined from a linear fit of peak times relative to the first recruited (index) electrode versus distance to the index in mm. The speed at which the low-frequency ictal discharges are distributed across the MEA was calculated from the maximum latency between negative peaks of each discharge; mean values with 95% confidence intervals were determined for a sample of 100 early-stage discharges per seizure ( Fig. 4 ). Spike-local field potential correlation Two second samples of pre-recruitment, post seizure onset time periods ('early') and post-recruitment ('late') were determined per channel for patients C5 and C7. Equivalent samples for patients C3 and C4 were selected immediately after seizure onset and immediately before seizure offset. Unit times were plotted circularly versus the instantaneous low-frequency phase. During a seizure, the low-frequency signal reflects synchronous, high amplitude rhythmic activity at a dominant frequency that gradually evolves over the course of the ictal event ( Fig. 3 ). Therefore, we calculated instantaneous phase from the wideband (2–50 Hz) Hilbert transform, as the phase at each time point is mainly determined by the predominant frequency. The correlation between spike timing and LFP phase was determined using the Rayleigh Z statistic. Significance levels were calculated using a bootstrap procedure: multiunit activity was circularly shifted relative to LFP by a random time interval between 0 and 10 s. The 95th percentile of the Rayleigh Z statistic for 10,000 trials was determined as the per-channel threshold for significance ( Figs 5 and 6 ). Coherence FIELDTRIP ( http://fieldtrip.fcdonders.nl/ ) software was used to calculate the weighted phase lag index, a coherence measure computed across trials from the imaginary component of the cross power spectrum [42] . This measure eliminates contributions from zero phase lag signals that could potentially be attributed to volume conduction. Postprocessed MEA LFP (downsampled to 1 kHz) were divided into trials defined by a sliding window 1 s in duration that advanced through the recording in 8 ms increments, then grouped into consecutive blocks of 20 trials, yielding a stepsize of 160 ms per block. The 2–30 Hz mean of the squared weighted phase lag index was calculated for each channel pair and trial block, for early and late seizure stages as described above. Seizure stereotypy Spearman correlation of LFP and multiunit activity for a given channel across seizures was calculated for those patients in whom multiple seizures were recorded (C2, C3, C4 and C5). Each seizure was divided into 100 equal duration segments, and both the number of multiunit spikes and sum (log (instantaneous 2–50 Hz amplitude)) (Hilbert transform) was calculated for each segment; data were smoothed using a moving average filter. Channels with less than 12 spikes s −1 over the course of the seizure were excluded from the multiunit activity calculations, to avoid the potential for sample bias due to artificially high variance from low spike rates. How to cite this article: Schevon C.A. et al . Evidence of an inhibitory restraint of seizure activity in humans. Nat. Comm. 3:1060 doi: 10.1038/ncomms2056 (2012).